Vortex magnetic structure in framboidal magnetite reveals existence of water droplets in an ancient asteroid The majority of water has vanished from modern meteorites, yet there remain signatures of water on ancient asteroids. How and when water disappeared from the asteroids is important, because the final fluid-concentrated chemical species played critical roles in the early evolution of organics and in the final minerals in meteorites. Here we show evidence of vestigial traces of water based on a nanometre-scale palaeomagnetic method, applying electron holography to the framboids in the Tagish Lake meteorite. The framboids are colloidal crystals composed of three-dimensionally ordered magnetite nanoparticles and therefore are only able to form against the repulsive force induced by the surface charge of the magnetite as a water droplet parches in microgravity. We demonstrate that the magnetites have a flux closure vortex structure, a unique magnetic configuration in nature that permits the formation of colloidal crystals just before exhaustion of water from a local system within a hydrous asteroid. The formation of the Solar System 4.6 billion years ago through the collapse of a cold molecular cloud was accompanied by many processes, including the evaporation and condensation of cosmic grains, their accretion into the smaller bodies of the Solar System and their modification in asteroids. Meteorites, debris sourced from larger cosmic bodies, such as asteroids, preserve evidence of the history of the Solar System. For instance, the signature of water in ancient asteroids has been observed in meteorites as veins of hydrothermally deposited minerals [1] or as water trapped in salt crystals [2] . The Tagish Lake meteorite, which fell at 16:43 on 18 January 2000 in southwestern Yukon, Canada, is a unique Type 2 carbonaceous chondrite, with affinities to CI and CM groups [3] , [4] , that may have originated from a D-type asteroid located in the middle of the asteroid belt [5] . This meteorite experienced negligible alteration and minimal contamination as a result of its rapid recovery after falling to Earth [4] . Abundant micrometre-sized polyhedral particles of magnetite are distributed in the matrix of the meteorite, together with clay minerals such as serpentine and saponite [3] , [4] . This paragenesis suggests that these minerals were formed by an aqueous process [6] , and many models for the evolution of type 2 carbonaceous chondrites have been proposed [3] , [7] . Recently, some framboidal magnetites in the Tagish Lake meteorite were recognized as colloidal crystals that consist of three-dimensionally assembled magnetites with diameters of 110–680 nm (ref. 8 ). The remanent magnetization of rocks and minerals is very sensitive to the chronology of their formation and to the temperature regimes that they have experienced [9] . The magnetization of the Tagish Lake meteorite has already been studied in bulk, and it has been reported that multidomain magnetites with a grain size of 4–9 μm make a major contribution to the magnetic properties [10] and that natural remanent magnetization persists at levels of up to 30 mT, suggesting that the magnetite formed in a weak magnetic field [11] . Here we show the occurrence of signatures of water originally present in the parent body based on a palaeomagnetic study of magnetite nanoparticles (resolution ~6 nm) isolated from colloidal crystals in the Tagish Lake meteorite. The study is performed by means of electron holography, a technique that permits the visualization of nanometre-scale magnetic properties with a transmission electron microscope (TEM; Supplementary Fig. S1 and Supplementary Note 1 ). 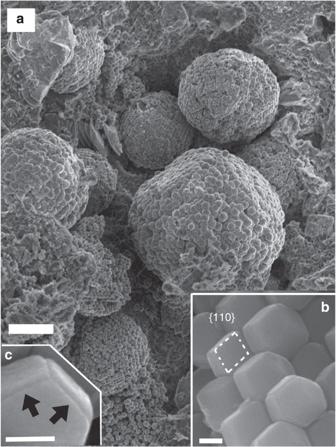Figure 1: SEM image of colloidal crystals of magnetite in the Tagish Lake meteorite. (a) The accelerating voltage of the scanning electron microscope (SEM) was 3.0 kV and the working distance was 8.8 mm. The scale bar is 1 μm. The insets are higher-magnification SEM images showing (b) a well-ordered colloidal crystal with a face-centered cubic structure and a rhombic–dodecahedral shape bounded only by {110} faces of the constituent particles and (c) notches along the crest indicated by arrows. The scale bars in (b) and (c) are 100 nm. Refer to the study by Nozawaet al.8for detailed descriptions of colloidal magnetite. Separation of magnetite nanoparticles from the meteorite Figure 1 shows a micrograph of an example of one of the colloidal crystals. Each colloidal crystal consists of 10 3 –10 4 magnetite nanoparticles, each of which is a single crystal, arranged with crystallographic coherence so that the magnetite nanoparticles behave as single atoms. The Tagish Lake sample was dispersed in ethanol with an ultrasonic generator and the resulting meteorite particles were dropped onto an amorphous carbon film supported by a TEM grid. The sample was loaded onto the magnetic field-free sample stage of the specially designed electron-holography TEM. In our current study, we were scrupulous in ensuring that the samples were not exposed to any artificial magnetic field at any stage during the experiments. Figure 1: SEM image of colloidal crystals of magnetite in the Tagish Lake meteorite. ( a ) The accelerating voltage of the scanning electron microscope (SEM) was 3.0 kV and the working distance was 8.8 mm. The scale bar is 1 μm. The insets are higher-magnification SEM images showing ( b ) a well-ordered colloidal crystal with a face-centered cubic structure and a rhombic–dodecahedral shape bounded only by {110} faces of the constituent particles and ( c ) notches along the crest indicated by arrows. The scale bars in ( b ) and ( c ) are 100 nm. Refer to the study by Nozawa et al. [8] for detailed descriptions of colloidal magnetite. Full size image Many kinds of fragments from the meteorites were distributed on the TEM grid. To identify magnetite particles in a portion of a colloidal crystal efficiently, we selected magnetite particles (~190 nm in diameter) with a rhombic–dodecahedron morphology typical of framboidal magnetite [8] ( Fig. 2a ). As a result, the [1-10] plane of the selected particles was inevitably aligned in the direction parallel to that of the electron beam under TEM observation. 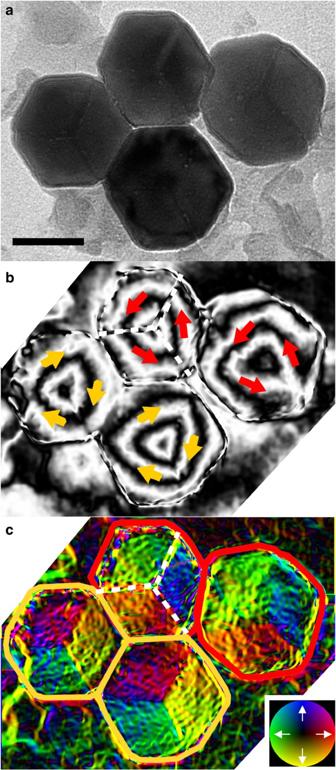Figure 2: TEM images of magnetite particles in a portion of a colloidal crystal. Images recorded by a Hitachi HF3300-EH with an acceleration voltage of 300 kV. (a) Bright field image. The scale bar is 100 nm. (b) Reconstructed phase distribution of (a) showing that each particle has a concentric circular magnetic field and a closed (that is, vortex) structure. The yellow and red arrows indicate clockwise and counterclockwise directions of the magnetization vectors in the magnetite particle, respectively. (c) Colour wheel map of the magnetization direction obtained from the reconstructed phase image. The white arrows show the direction of the magnetization direction. The colour changes in the profiles of the magnetite indicate the direction of the magnetization vectors; clockwise: yellow, counterclockwise: red. All the fragments of the colloidal crystals that we observed showed magnetization with both clockwise and counterclockwise magnetic moments. Figure 2: TEM images of magnetite particles in a portion of a colloidal crystal. Images recorded by a Hitachi HF3300-EH with an acceleration voltage of 300 kV. ( a ) Bright field image. The scale bar is 100 nm. ( b ) Reconstructed phase distribution of ( a ) showing that each particle has a concentric circular magnetic field and a closed (that is, vortex) structure. The yellow and red arrows indicate clockwise and counterclockwise directions of the magnetization vectors in the magnetite particle, respectively. ( c ) Colour wheel map of the magnetization direction obtained from the reconstructed phase image. The white arrows show the direction of the magnetization direction. The colour changes in the profiles of the magnetite indicate the direction of the magnetization vectors; clockwise: yellow, counterclockwise: red. All the fragments of the colloidal crystals that we observed showed magnetization with both clockwise and counterclockwise magnetic moments. Full size image Visualization of the magnetic configuration of magnetite The TEM has an additional sample stage located 10 cm above the objective lens. The size of this gap permits the sample stage to be maintained in a very weak magnetic field of <17 μT, which is weaker than the earth’s magnetic field, in the direction opposite to the electron beam, thereby ensuring that the original magnetic properties of the meteoritic sample were retained. We visualized the magnetic structures in the individual particles by electron holography. The information obtained by electron holography generally contains details of both the magnetic flux and the internal electric potential of the sample; these cannot be separated in a single hologram. To retrieve the magnetic information, we prepared two kinds of hologram for each meteorite sample. The first hologram was taken from one side of the sample and the second was recorded from the other side after inverting the sample. The internal potential was removed by subtraction of the phase changes reconstructed from the two holograms ( Supplementary Fig. S2 ). Figure 2b shows a contour-line map of the reconstructed phase image, corresponding to the magnetic flux distribution. The arrows indicate the direction of the in-plane magnetization vectors in the magnetite particle. Figure 2c shows a colour wheel map of the magnetization obtained from the phase image. A comparison of these experimental images with simulated electron holographic images ( Supplementary Figs S3 and S4 ) showed that the particles had an in-plane magnetization of ~0.6 T. Although this value is close to the saturated magnetization value of magnetite [12] , this is not a result of exposure to a strong magnetic field but is the result of the presence of a vortex structure. The electron holographic images clearly show that, unlike common magnetite, each particle has a flux closure vortex structure [13] . The external magnetic fields of the particles are below the detection limit of h /(30 e ) Wb, where h is Planck’s constant and e is the elementary charge. It is possible that the magnetization in the centre of the vortex structure contains a stray field [14] , [15] and that its interactions may have contributed to the formation of the colloidal crystal. However, we did not find any detectable stray field or any evidence of its interaction with nearby magnetites. Exposure experiments in magnetic fields Magnetic configurations can be affected by the direction and strength of external magnetic fields and by the arrangements of the magnetic crystals [16] . To observe the collective magnetic behaviour of colloidal crystals of magnetite, we applied a vertical magnetic field and a strong ‘in-plane’ magnetic field sequentially to the magnetite particles in two portions of the colloidal crystals. 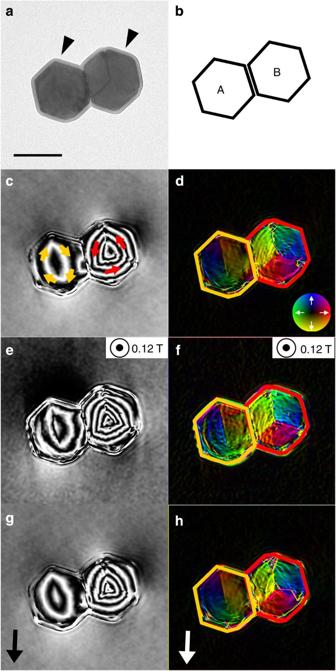Figure 3: TEM images of magnetite particles in exposure experiments into magnetic fields. Images of a part of a framboidal magnetite from the Tagish Lake meteorite were recorded by a Hitachi HF3300-EH with an acceleration voltage of 300 kV. (a) Bright field image after deposition of amorphous carbon on the sample to avoid rotation during a series of experiments. Two triangles show the carbon layer of a brighter contrast than magnetite particles. (b) Schematic showing the discrimination of individual magnetite particles with labels A and B. (c) Reconstructed phase distribution of (a) in non-magnetic field after subtracted internal potential. Each particle shows a concentric circular magnetic field and a closed (that is, vortex) structure. The yellow and red arrows indicate the directions of the magnetization vectors in the magnetite particle; yellow: clockwise (particle A); red: counterclockwise (particle B). (d) Colour wheel map of the magnetization direction obtained from the reconstructed phase image (c). The white arrows in the wheel show the direction of the magnetization. Colour changes in the profiles of the magnetite (d,fandh) indicate the direction of the magnetization. (e) Reconstructed phase distribution of the magnetite particles in a magnetic field of 0.12 T to the opposite direction of electron beam after subtracted internal potential showing that each particle still has a concentric circular magnetic field and a closed (that is, vortex) structure. (f) Colour wheel map of the magnetization direction obtained from the reconstructed phase image (e). (g) Reconstructed phase distribution of the magnetite particles in non-magnetic field, but after exposure the sample to a strong ‘in-plane’ magnetic field of 1.9 T for 5 min to the direction indicated by an arrow. Internal potential has been subtracted. Both particles still have a concentric circular magnetic field and a closed (that is, vortex) structure. (h) Colour wheel map of the magnetization direction obtained from the reconstructed phase image (g). The scale bar in (a) is 200 nm. Figure 3 and Supplementary Fig. S5 show the resulting TEM images of portions containing two and six magnetite particles, respectively. Initially, we recorded the original magnetic configuration of the samples before they were exposed to the magnetic field ( Fig. 3c,d and Supplementary Fig. S5c,d ). All the particles had a vortex structure, but particles A, C and H were tilted from the direction of the electron beam. We then applied a magnetic field of 0.12 T in the opposite direction to the electron beam, and we recorded the holograms of the particles in the magnetic field ( Fig. 3e,f and Supplementary Fig. S5e,f ). One contour line of B ( Fig. 3f ) increased and the colour wheel maps for all the magnetites shown in Fig. 3f and Supplementary Fig. S5f became brighter than the corresponding maps before exposure. The degree of the phase tilt indicated a quantitative increase of ~18% in the in-plane moment of magnetization of the magnetites. This showed that the direction of the vortex configuration was tilted away from the in-plane direction toward the direction of the electron beam. Figure 3: TEM images of magnetite particles in exposure experiments into magnetic fields. Images of a part of a framboidal magnetite from the Tagish Lake meteorite were recorded by a Hitachi HF3300-EH with an acceleration voltage of 300 kV. ( a ) Bright field image after deposition of amorphous carbon on the sample to avoid rotation during a series of experiments. Two triangles show the carbon layer of a brighter contrast than magnetite particles. ( b ) Schematic showing the discrimination of individual magnetite particles with labels A and B. ( c ) Reconstructed phase distribution of ( a ) in non-magnetic field after subtracted internal potential. Each particle shows a concentric circular magnetic field and a closed (that is, vortex) structure. The yellow and red arrows indicate the directions of the magnetization vectors in the magnetite particle; yellow: clockwise (particle A); red: counterclockwise (particle B). ( d ) Colour wheel map of the magnetization direction obtained from the reconstructed phase image ( c ). The white arrows in the wheel show the direction of the magnetization. Colour changes in the profiles of the magnetite ( d , f and h ) indicate the direction of the magnetization. ( e ) Reconstructed phase distribution of the magnetite particles in a magnetic field of 0.12 T to the opposite direction of electron beam after subtracted internal potential showing that each particle still has a concentric circular magnetic field and a closed (that is, vortex) structure. ( f ) Colour wheel map of the magnetization direction obtained from the reconstructed phase image ( e ). ( g ) Reconstructed phase distribution of the magnetite particles in non-magnetic field, but after exposure the sample to a strong ‘in-plane’ magnetic field of 1.9 T for 5 min to the direction indicated by an arrow. Internal potential has been subtracted. Both particles still have a concentric circular magnetic field and a closed (that is, vortex) structure. ( h ) Colour wheel map of the magnetization direction obtained from the reconstructed phase image ( g ). The scale bar in ( a ) is 200 nm. Full size image The sample was then moved from the specially designed sample stage to an ordinary sample stage in the same TEM, and the sample was rotated 90° to apply a strong in-plane magnetic field in the direction shown by the arrows in Fig. 3g,h and Supplementary Fig. S5g,h . After exposure of the sample to a magnetic field of 1.9 T for 5 min, the sample was returned to the specially designed non-magnetic sample stage and a hologram was recorded. Note that the electron hologram cannot be recorded on the ordinary common sample stage during exposure to the strong in-plane magnetic field. Figure 3g,h and Supplementary Fig. S5g,h show micrographs of the resulting magnetite particles taken in the absence of a magnetic field. The strength of their magnetization was increased by only 2%, which is within the limits of error. Therefore, the magnetic configuration of the magnetite particles had reverted to the initial configuration. The only difference was in the direction of the vortex magnetization of particle E. As the magnetite particles were fixed by the deposition of the carbon film, the change from the clockwise direction of the vortex before exposure to the in-plane magnetic field to a counterclockwise direction after exposure is not a result of physical rotation of the particle but is caused by rearrangement of its magnetic moment. The magnetization during exposure to the in-plane magnetic field would be expected to be in the same direction as the field; unfortunately, however, we were unable to observe this. This experiment shows that the stable magnetic structure of a framboidal magnetite is characterized by vortex magnetization and that framboidal magnetites do not have an external magnetic stray field and do not interact magnetically with each other even after exposure to a strong magnetic field. The surface layer of the magnetite The surfaces of the magnetite particles might contain residues from their mother solution. When we used high-resolution TEM to examine the surface layer, we found that many of the magnetites had an amorphous surface layer 0–3 nm thick. 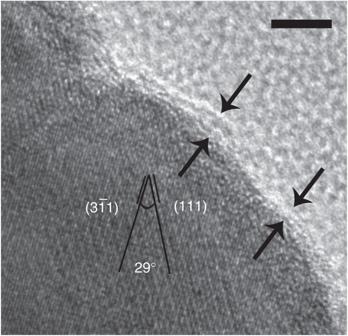Figure 4: High-resolution TEM image of a surface of magnetite. Image recorded by a JEOL JEM-2100F with an acceleration voltage of 300 kV. Crossed lattice fringes of 0.485 nm (corresponding to (111)) and 0.253 nm (corresponding to (3-11)) at an angle of 29°, corresponding to magnetite, are visible. The pairs of arrows indicate an amorphous layer on the surface of the magnetite particle. The scale bar is 5 nm. Figure 4 shows an example of such an amorphous surface layer delineated by pairs of arrows. Some magnetites have lattice fringes at the ends of the particles, showing that they have no surface layer. Energy-dispersive X-ray analysis (EDX) spectra recorded at several locations, from the surface to the centre, for more than 10 particles, showed no significant evidence of enrichment by any elements other than iron, oxygen, carbon and copper ( Fig. 5 ). Elemental mapping also showed no evidence of condensation of residues on the surface of a magnetite ( Fig. 6 ). The surface layer might therefore consist of carbonaceous materials. Figure 4: High-resolution TEM image of a surface of magnetite. Image recorded by a JEOL JEM-2100F with an acceleration voltage of 300 kV. Crossed lattice fringes of 0.485 nm (corresponding to (111)) and 0.253 nm (corresponding to (3-11)) at an angle of 29°, corresponding to magnetite, are visible. The pairs of arrows indicate an amorphous layer on the surface of the magnetite particle. The scale bar is 5 nm. 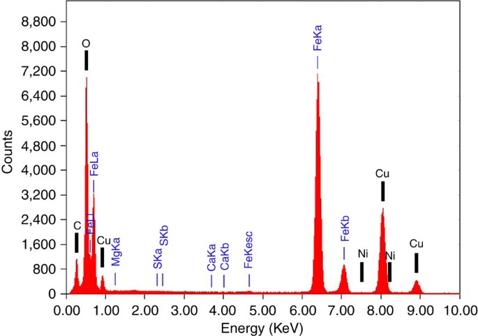Figure 5: EDX spectrum of a framboidal magnetite. The sample shown inFig. 6was analysed using a JEOL EX-2300. Peaks labelled C and Cu originate from the amorphous carbon substrate and the TEM grid, respectively. No peaks other than that of iron originating from the magnetite were detected, even when the electron beam was focused on other locations in the particles. Full size image Figure 5: EDX spectrum of a framboidal magnetite. The sample shown in Fig. 6 was analysed using a JEOL EX-2300. Peaks labelled C and Cu originate from the amorphous carbon substrate and the TEM grid, respectively. No peaks other than that of iron originating from the magnetite were detected, even when the electron beam was focused on other locations in the particles. 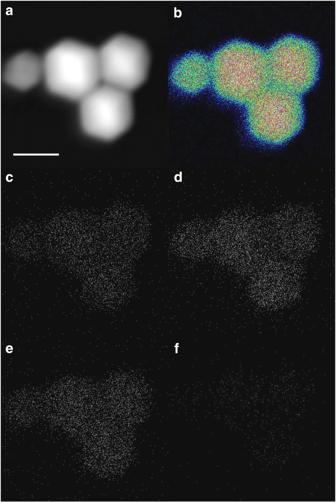Figure 6: Electron micrograph and elemental mapping images of magnetite. Images of a part of a framboidal magnetite from the Tagish Lake meteorite were recorded by scanning TEM (STEM) with a high-angle annular dark-field (HAADF) detector (JEM-2100 F) and an EDX spectrometer. (a) HAADF–STEM image. (b–f) Corresponding elemental mapping images for iron (b), calcium (c), magnesium (d), sulphur (e) and nickel (f). The scale bar in (a) is 200 nm. Full size image Figure 6: Electron micrograph and elemental mapping images of magnetite. Images of a part of a framboidal magnetite from the Tagish Lake meteorite were recorded by scanning TEM (STEM) with a high-angle annular dark-field (HAADF) detector (JEM-2100 F) and an EDX spectrometer. ( a ) HAADF–STEM image. ( b – f ) Corresponding elemental mapping images for iron ( b ), calcium ( c ), magnesium ( d ), sulphur ( e ) and nickel ( f ). The scale bar in ( a ) is 200 nm. Full size image The flux closure vortex structure observed here has been regarded as a pseudo-single-domain structure [17] . There is no report of any natural occurrence of such a vortex structure; however, a three-dimensional (3D) micromagnetic simulation predicted the existence of a uniformly magnetized single-domain vortex state for cubic structures with edge lengths of 70–140 nm (ref. 18 ). An electron holograph of a finely exsolved intergrowth of submicron magnetite blocks at a nanometre-scale demonstrated, for the first time, the presence of a vortex state arising from the interaction of magnetite blocks with single magnetic domain structure in a natural rock [19] . As the magnetic structures of ferromagnetic nanoscale materials depend on their geometry rather than on their intrinsic material properties [20] , [21] , the magnetic structure of framboidal magnetite should be directly related to the environment in which it was formed and to the processes from which the magnetite obtained it’s magnetization. As size increases, the magnetic structure of magnetite changes sequentially from a superparamagnetic state to a single domain, then to a vortex and eventually to a multidomain state. The corresponding transitional particle sizes, calculated from the local energy minimum states, are 20–50, ~70 and ~140 nm, respectively, if the particles are assumed to be cubic [18] . The volumes of the present particles are about 5–10 times larger than the volume for the transitional particle size between the vortex and multidomain states. Nevertheless, all the meteoritic magnetite particles showed a flux closure vortex configuration with threefold symmetrical domain walls that minimize their magnetostatic energy, which is increased by magnetic field leakage [17] . The characteristic shape with notches along the crest, as indicated by arrows in Fig. 1c , is also favourable for maintaining vortex magnetization [22] . The morphology of the crystal’s equilibrium form is an effort to minimize the total energy of the system. In the case of nanoparticles, surface free energies govern the morphology because of the large surface-to-volume ratio. Here the magnetostatic energy of the magnetic nanoparticles might be able to contribute to the determination of the morphology because of the significantly small total surface area (energy). When the magnetite particle has a magnetic domain wall, the energy disadvantage becomes of the order of 10 –17 J, which is of a similar magnitude to the increase in surface free energy arising from formation of the notches (See Methods). This may be the first example in which the morphology of a crystal has been shown to be affected by its internal magnetostatic energy [23] . Magnetite framboids are abundant in matrices and clasts in association with serpentine, saponite, carbonates and pyrrhotite in the carbonate-poor lithology of the Tagish Lake meteorite. This lithology provides evidence of temperature elevations above the freezing point of water as a result of highly energetic impacts [24] and/or the decay heat of radiogenic aluminium-26 (ref. 25 ). During aqueous alteration, Ca, Al, Si-rich mesostasis glass, anhydrous silicates such as olivine and pyroxene and Fe metal inclusions in chondrules and fine silicates in the matrix are altered and upon hydration they released cations such as Mg, Ca and Fe into the solution. Magnesium and calcium in solution initially precipitated as carbonate during alterations in the aqueous environment of the asteroid. The resulting solution then became relatively enriched in iron ions, which favoured the direct precipitation of magnetite [26] . The presence of saponite and an analysis of the organic compounds present imply that the pH of the solution was >7 and that the upper limit of the alteration temperature was 150 °C (refs 26 , 27 ). Lower temperatures would tend to broaden the region in which magnetite is stable in an iron-sulphur-oxygen system [28] . As many altered chondrules and phyllosilicate aggregates have a sulphide-enriched rim, sulphides are expected to result from late-stage mineralization. Some magnetite forms a thin rim around pyrrhotite, suggesting that the magnetite has replaced the pyrrhotite, that is, it is a pseudomorph [3] . If the magnetite was formed from a precursor, the solution condition must have changed from relatively sulphur-rich to oxygen-rich with respect to the metallic iron. This environmental change might have occurred during initial formation of pyrrhotite before the formation of magnetite. As a result, a lithology of pyrrhotite surrounded by magnetite, as shown by Zolensky et al. would be formed [3] . However, it would be difficult to eliminate all sulphur from the system in a solution. After sublimation of water, sulphur could leach from pyrrhotite and be replaced by oxygen. Colloidal crystals would then be formed from pyrrhotite. In such a case, fine microstructures of the polyhedral morphology would not be preserved and the magnetite should contain voids at the centre of the particles as a result of volume reduction and diffusion of iron from inside to outside to form oxides [29] , as reported for terrestrial magnetites formed from pyrite [30] . Furthermore, framboidal sulphides such as pyrrhotite, pentlandite or greigite have never been found in meteorites. The pyrrhotite and pentlandite in the Tagish Lake meteorite contain nickel atoms in amounts of ~10 and 50% with respect to iron [3] . Nevertheless, EDX analysis spectra of framboidal magnetite did not show a significant peak for nickel (<1%). If framboidal magnetite is a pseudomorph of these sulphides, the magnetite should contain nickel, which should form a solid solution with trevorite (NiFe 2 O 4 ). Greigite has the same crystallographic structure as magnetite and its volume is similar. However, greigite can be excluded as a precursor, because abundant greigite has not been found in meteorites and there are no realistic conditions for the transformation of a greigite-rich lithology into a lithology that is rich in magnetite accompanied by pyrrhotite and pentlandite. The unique morphologies, in the form of several kinds of polyhedron, and the perfection of the framboidal magnetite particles suggest that the colloidal crystals must have formed by direct precipitation from solution. We therefore believe that the framboidal magnetite was not formed by oxidation of a precursor. The existence of colloidal crystals provides further information about the solution environment. 3D arrangements of hard spheres (colloidal crystals) in a solvent have been studied extensively because they provide a model for nucleation and growth of crystal in general [31] , [32] and they have potential for use as materials such as photonic crystals [33] . Supersaturation is a prerequisite for the formation of colloidal crystals, just as in the case of normal crystallization from a solution [34] , [35] . As colloidal crystals are stabilized by a repulsive force, the density of magnetite particles in a solution must be sufficiently high in a limited solution to overcome this force, as explained by the Derjaguin–Landau–Verwey–Overbeek (DLVO) theory [36] , [37] . If the magnetite particles were typical magnets, they would have readily coagulated into a single grain as a result of the strong attractive magnetic interactions and they would not have produced a well-ordered colloidal structure [38] . Higher surface charges and lower ionic concentrations favour the formation of colloidal crystals. The surface charge of magnetite in aqueous solutions becomes zero in the pH range of 5.4–6.8 at 30–90 °C (refs 39 , 40 ). This pH range is lower than the thermochemically calculated value of 7–12 for the bulk solution during the main aqueous-alteration stage in parent bodies of carbonaceous chondrites [41] , [42] . The difference in pH values can be explained by adsorption of ions such as Ca 2+ and Mg 2+ at levels of 10 –14 –10 –15 mol m –2 onto the surface of the magnetite [43] . The concentration of these ions in their mother solution would then be of the order of 10 –3 –10 –4 mol. EDX analysis did not show any evidence of sediments on the surface layer but they did imply the deposition of carbonaceous materials ( Figs 5 and 6 , and Supplementary Note 2 ). As a colloidal crystal is formed in the presence of a repulsive force, it is necessary to use a system enclosed within a container to obtain colloidal crystals in a laboratory. The required volume fraction of colloidal particles dependent on the Debye screening length must exceed 50% (refs 31 , 34 ). However, the magnetite particles found in the hollows of various carbonaceous chondrites, including most of those from Tagish Lake meteorite, are not aligned three-dimensionally. Furthermore, the magnetite particles have a wide size distribution [3] , [44] . This may be a result of heterogeneous nucleation on the hollow surfaces of the surrounding minerals. The uniformity of the size distribution and the similar morphology of the framboidal magnetite particles in each of the colloidal crystals suggest that they were formed through homogeneous nucleation from a highly supersaturated isolated solution in a single nucleation event. The very low gravitational force present in small asteroids or close to the centre of asteroids permit the formation of closed systems in the form of droplets stabilized by the effects of surface tension, which overcomes any gravitational forces, as shown in Fig. 7 . The formation of such droplets eliminates the need for the presence of a container. To preserve the homogeneity of the solution in droplets to achieve a single nucleation event in a high degree of supersaturation, the timescale for sublimation of water from the solution must have been longer than that for diffusion of ions, thereby resulting in a relatively high rate of magnetite nucleation once appropriate conditions were achieved within each droplet. If the nucleation rate in the solution was low, as the result of a low degree of supersaturation, and nucleation was driven by external factors, such as shocks caused by multiple collisions of asteroids within a short period, single crystals or very few crystals with wide size distributions would probably have formed framboids such as those observed in various carbonaceous chondrites [3] , [44] . Therefore, the framboidal magnetite nanoparticles could not have been formed during the main stage of massive aqueous alteration, but were probably formed later from the very last droplets of aqueous solution remaining in the meteorite parent body after the bulk of the fluid reservoir had been lost from the system. 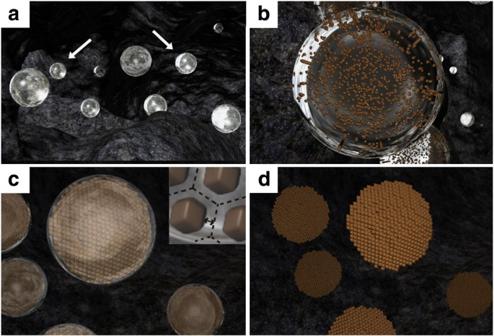Figure 7: Formation process of colloidal magnetite crystals in the Tagish Lake meteorite. (a) Many droplets of supersaturated solution, which can form as a result of shaking due to collision24, are distributed in crevices of the parent asteroid. (b) Magnetite particles (brown dots) nucleate simultaneously to produce a uniform size and shape in each droplet. (c) The colloidal particles arrange by repulsive force to form a colloidal crystal in the solution. To overcome this force, the density of magnetite particles in a solution must be sufficiently high in a limited solution. The diameter of each droplet is ~25% larger than that of the final product seen in (d). The increase in the volume fraction of magnetite can be achieved through evaporation of water from (b) to (c). Enlarged image of the inside of a droplet (inset in (c)) shows that the particles cannot approach one another more closely than the Debye screening length (double ended black arrow) due to the presence of a screened coulomb potential, as explained by the DLVO theory36,37. Only in the case of equivalent distances between particles and the Debye screening length of each particle can they arrange and make a colloidal crystal. (d) Further evaporation reduces the inter-particle spaces until the colloidal crystals are stabilized by desiccation. Figure 7: Formation process of colloidal magnetite crystals in the Tagish Lake meteorite. ( a ) Many droplets of supersaturated solution, which can form as a result of shaking due to collision [24] , are distributed in crevices of the parent asteroid. ( b ) Magnetite particles (brown dots) nucleate simultaneously to produce a uniform size and shape in each droplet. ( c ) The colloidal particles arrange by repulsive force to form a colloidal crystal in the solution. To overcome this force, the density of magnetite particles in a solution must be sufficiently high in a limited solution. The diameter of each droplet is ~25% larger than that of the final product seen in ( d ). The increase in the volume fraction of magnetite can be achieved through evaporation of water from ( b ) to ( c ). Enlarged image of the inside of a droplet (inset in ( c )) shows that the particles cannot approach one another more closely than the Debye screening length (double ended black arrow) due to the presence of a screened coulomb potential, as explained by the DLVO theory [36] , [37] . Only in the case of equivalent distances between particles and the Debye screening length of each particle can they arrange and make a colloidal crystal. ( d ) Further evaporation reduces the inter-particle spaces until the colloidal crystals are stabilized by desiccation. Full size image Sample preparation The Tagish Lake meteorite has two lithologies: a dominant carbonate-poor lithology and a less-abundant carbonate-rich lithology [3] . Magnetite is predominantly distributed in the carbonate-poor lithology rather than in the carbonate-rich lithology and it is present as framboids, placquettes and euhedral single grains. After gently grinding a small piece of the Tagish Lake meteorite with carbonate-poor lithology, the powder was poured into a 10 ml bottle filled with ethanol and the mixture was agitated by ultrasound. A 5–10 μl aliquot of the suspension was removed with a pipette and dropped onto a thin film of amorphous carbon supported on a standard copper grid of a TEM. The sample was loaded into the specially designed electron-holography TEM that had an additional sample stage maintained in a magnetic field-free environment (<17 μT). As many kinds of particle were present on the grid, it was very difficult to identify particles of magnetite. We therefore selected a cluster of particles with the typical rhombic–dodecahedral morphology of framboidal magnetite [8] to permit efficient identification of a magnetite particle as part of the framboidal magnetite. As a result, the particles under TEM observation were inevitably oriented in the [1-10] direction. Analytical method for determining the magnetic component To observe the distribution of magnetic flux in a sample of non-uniform thickness, such as the magnetite particles described in this paper, the phase information pertaining to the electric inner potential of the sample has to be removed from the reconstructed object wave. When an electron wave penetrates a magnetic sample with domains, as shown in Supplementary Fig. S2a , magnetic (pink) and inner potential (sky blue) components are detected together as a reconstructed phase. Note that these two components cannot be separated in a single image. However, if the sample is inverted and the electron wave penetrates from the other side, as shown in Supplementary Fig. S2b , the sign of the phase change arising from the magnetic component becomes opposite to the original, because the direction of the Lorentz force is opposite, whereas the phase change arising from the inner potential component remains the same. The inner potential can therefore be removed by subtracting the reconstructed phase of Supplementary Fig. S2b from that of Supplementary Fig. S2a . As a result we can obtain the phase change arising from the magnetic component (pink), as shown in Supplementary Fig. S2c ; note that the amplitude of this phase change is double of that obtained from a single image. We recorded two experimental holograms of each magnetite particle (see Fig. 2a ) in this way and we reconstructed the twofold amplified phase image. The contour-line map of the reconstructed phase image corresponds to the magnetic flux distribution ( Fig. 2b ). To generate the colour-wheel map that shows the magnetic domain structures, x and y differential values of the phase image were calculated and the vector directions were displayed as different colours ( Fig. 2c ). Simulation of the electron-holography image We performed a simulation of the electron-holography image to evaluate the magnetic flux distribution in the magnetite particles ( Fig. 2b and c ). We assumed that the magnetite particle is spherical with a diameter of 190 nm. We also assumed that the particle has three domains uniformly separated by walls parallel to the z axis and that the magnetization vectors are in the x – y plane of each domain, as shown in Supplementary Fig. S3a (clockwise closure domains) and Supplementary Fig. S4a (counterclockwise closure domains). The spherical particle is regarded as a 3D assembly of a large number of small magnetic dipoles ( Supplementary Figs S3b and S4b ). We then calculated the phase distribution arising from each individual dipole (0.63 nm cube) with the algorithm reported by Hirayama et al. [45] and by Yamamoto et al. [46] , and we integrated all the phase values, taking into consideration the thickness change and the magnetic domains of the particle [47] , [48] . Supplementary Figs S3c and S4c show the resulting phase distribution projected onto the x – y plane. The sign of the phase in Supplementary Fig. S3c is opposite to that in Supplementary Fig. S4c because the direction of the closure vortex is opposite. Supplementary Figs S3d and S4d are the twofold amplified phase contour maps showing the distribution of magnetic flux. Supplementary Figs S3e and S4e show the corresponding colour-wheel maps obtained from the each phase image. The contour maps and the colour-wheel maps are similar to those obtained experimentally for the magnetite particles, as shown in Fig. 2b,c . The magnetization used in this simulation was 0.60 T, the accepted value for bulk magnetite. Balance between surface and magnetic domain wall energies The formation of notches along the 24 80–90-nm-long crests of the magnetite particles results in an increase in their total surface area by about 1 × 10 –14 m 2 , if the width of each crest is 0.42 nm, as estimated from the size of the unit cell of magnetite. As the surface free energy of magnetite [49] is 6.1 × 10 –2 J m –2 , the total surface energy increase is ~5 × 10 –17 J. If a magnetite particle with 85 nm in radius produces a magnetic domain wall in its centre, it will obtain an energy disadvantage of ~2 × 10 –17 J from the magnetic domain wall energy [50] of 9.3 × 10 –14 J m –2 . This very rough estimation suggests that the energy disadvantages obtained from forming notches or forming magnetic domain walls are of similar magnitude and therefore that the morphology of the crystal might be affected by the magnetic energy. How to cite this article: Kimura, Y. et al. Vortex magnetic structure in framboidal magnetite reveals existence of water droplets in an ancient asteroid. Nat. Commun. 4:2649 doi: 10.1038/ncomms3649 (2013).